Transmembrane anion transport mediated by halogen-bond donors In biology and chemistry, the transport of anions across lipid bilayer membranes is usually achieved by sophisticated supramolecular architectures. Significant size reduction of transporters is hampered by the intrinsically hydrophilic nature of typical anion-binding functionalities, hydrogen-bond donors or cations. To maximize the atom efficiency of anion transport, the hydrophobic nature, directionality, and strength of halogen bonds seem promising. Unlike the ubiquitous, structurally similar hydrogen bonds, halogen bonds have not been explored for anion transport. Here we report that transport across lipid bilayers can be achieved with small perfluorinated molecules that are equipped with strong halogen-bond donors. Transport is observed with trifluoroiodomethane (boiling point=−22 °C); that is, it acts as a 'single-carbon' transporter. Contrary to the destructive action of small-molecule detergents, transport with halogen bonds is leakage-free, cooperative, non-ohmic and highly selective, with anion/cation permeability ratios <37. Ion transporters regulate ion concentrations across membranes. In biology, anion transport is usually achieved by very large transmembrane proteins with multiple anion-binding sites for cooperative transport at high selectivity and speed. The creation of synthetic anion transporters has attracted attention owing to possible applications in the materials sciences (for example, as sensors and photosystems) and in medicine (possible treatment of channelopathies, for example, cystic fibrosis) [1] , [2] , [3] , [4] , [5] , [6] , [7] , [8] , [9] , [10] , [11] , [12] , [13] . Anion transport is usually achieved by hydrogen bonding and ion pairing. Recent synthetic anion transporters that operate this way include elegant variations of the natural product prodigiosin, isophthalates with intramolecular aminoxy turns in their sidechains, amphiphilic biscatechols, phospholipids with ureas at the end of one tail, cholate scaffolds with urea sidechains at their hydrophilic face, peptide–lipid hybrids or artificial β-barrels [1] , [2] , [3] , [4] , [5] , [6] . Anion transport mediated by hydrogen bonds or ion pairs has also been realized with macrocycles such as calixpyrroles, phosphate-linked oligosaccharides or the classical cyclodextrins [1] , [2] , [3] , [4] , [5] , [6] . Of highest importance in many biological systems, anion-macrodipole interactions have been engineered only recently into a synthetic anion transport system composed of stacked urea/amide macrocycles [7] . Successful transport with anion-π interactions [10] , [11] , finally, provided the first example for the functional relevance of these less recognized interactions. Moreover, this finding expanded number and nature of the interactions available to design and synthesize anion transporters beyond biological precedence. Here we add halogen bonds to this collection. Halogen bonds form between nucleophilic acceptors, such as anions, and highly localized positive-charge density on halogen atoms appearing on the side opposite to the covalent bond [13] , [14] , [15] , [16] , [17] , [18] , [19] , [20] , [21] , [22] . They are most prominent with iodine atoms but occur, to a lesser extent, also with the less polarizable bromine, chlorine, and even fluorine ( Fig. 1a ) [14] . Their strength increases with the hydrophobicity of non-competitive solvents [15] . 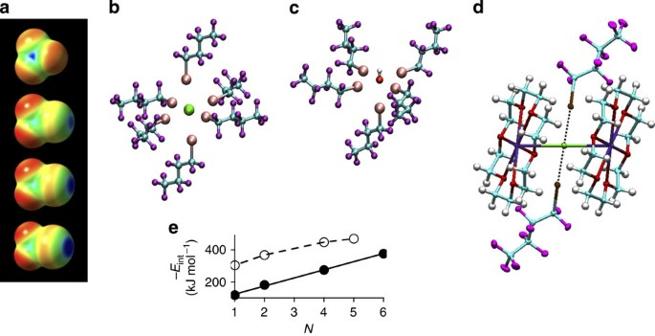Figure 1: DFT optimized structures of halogen-bonded transport systems and crystal structure. (a–d), Electrostatic potential surfaces (a) of, top to bottom, CF4, CF3Cl, CF3Br and CF3I (blue, +105, green +65, red −25 kJ mol−1, isovalue 0.001 a.u.), ball-and-stick models of chloride (b) and hydroxide (c) bound to, respectively, six and five perfluoro-1-iodobutanes 4 obtained by DFT simulations, and (d) crystal structure of chloride bound to two transporters 4 and potassium counterions bound to 18-crown-6 (C, cyan; H, white; O; red; F, magenta; I, pink; Cl−, green; K+, violet). (e) Chloride (filled circle) and hydroxide (empty circle) binding energy (Eint) in kilojoule per mole (kJ mol−1) as a function of the numberNof transporters 4. Figure 1: DFT optimized structures of halogen-bonded transport systems and crystal structure. ( a–d ), Electrostatic potential surfaces ( a ) of, top to bottom, CF 4 , CF 3 Cl, CF 3 Br and CF 3 I (blue, +105, green +65, red −25 kJ mol −1 , isovalue 0.001 a.u. ), ball-and-stick models of chloride ( b ) and hydroxide ( c ) bound to, respectively, six and five perfluoro-1-iodobutanes 4 obtained by DFT simulations, and ( d ) crystal structure of chloride bound to two transporters 4 and potassium counterions bound to 18-crown-6 (C, cyan; H, white; O; red; F, magenta; I, pink; Cl−, green; K + , violet). ( e ) Chloride (filled circle) and hydroxide (empty circle) binding energy ( E int ) in kilojoule per mole (kJ mol −1 ) as a function of the number N of transporters 4. Full size image Routinely exploited in crystal engineering [14] , halogen bonds are attracting only recently some attention for rational drug design [16] , anion binding [17] , [18] and catalysis [19] , [20] . Whereas the special behaviour of molecular iodine (bp=184 °C) has been noticed early on [21] , [22] , contributions of organic halogen bonds to the transport of anion across lipid bilayer membranes have been suspected last year, for the first time [13] . However, their contribution to a less attractive anion/cation symport with multivalent calixarenes has never been fully confirmed. To experimentally demonstrate the functional relevance of halogen bonds for anion transport, we attempted to identify the smallest possible active molecules with little more than a halogen-bonding moiety. However, previous attempts to reduce size and sophistication of synthetic ion transporters have often resulted in inactivity or activities with nonspecific, undesirable characteristics. Most impressive are the destructive actions of small-molecule detergents such as hexafluoroisopropanol [12] . Examples for small molecules with hydrophilic hydrogen-bond donors/acceptors that are inactive include propanol, diethylether or anisole. Successful but less dramatic structural reductionism has occurred previously with thioureas as most hydrophobic hydrogen-bond donors [9] and naphthalenediimide transporters that operate with anion-π interactions [10] , [11] . Halogen bonds seemed particularly promising to reduce the size of anion transporters, because they can be considered as hydrophobic equivalents of hydrogen bonds (that is, directional and strong) [14] . Transporters that work with halogen bonds do not contain hydrophilic binding sites that have to be overcompensated with large hydrophobic domains. Moreover, the boiling point of transporters with halogen bonds can be very low. In the following, we report that halogen-bond donors as small as trifluoroiodomethane (bp=−22 °C) or, preferably, perfluoroiodohexane or tetrafluorodiiodobenzenes, can transport anions across bilayer membranes in a leakage-free, non-ohmic and highly selective manner. Molecular modelling and crystal structures A collection of 19 candidates 1 – 19 was targeted for anion transport experiments ( Fig. 2 ). For selected structures from this series, computational studies were made by density functional theory (DFT) at the M06L-L/6-311G** (geometry) [23] and M06-2X/6-311G** levels (binding) [24] in the 'membrane-mimetic' gas phase [10] . They revealed that chlorides can be encapsulated within a hydrophobic shell formed by up-to-six halogen-bonded ligands 4 in a quasi-octahedral geometry (−376.9 kJ mol −1 ; Fig. 1b ), whereas hydroxides can interact only with up-to-five (−469.5 kJ mol −1 ; Fig. 1c ). For chloride and hydroxide anions with increasing number of ligands 4 , the binding progressively increased ( Fig. 1e ). Ligand replacement by water molecules reduced anion binding to −302.8 kJ mol −1 and −386.0 kJ mol −1 , respectively, indicating that anion transport should occur in both cases with dehydration and follow an anti-Hofmeister selectivity ( Fig. 3c ) [25] . Weakening of the halogen bonds by defluorination as in iodohexane 5 and iodobenzenes 18 or substitution of iodine by bromine as in pentafluorobromobenzene 11 resulted in clearly weaker binding ( Fig. 2 ). 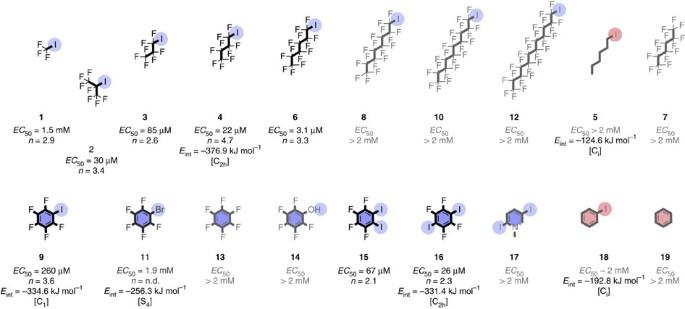Figure 2: Candidates tested for anion transport with halogen bonds. Effective concentrations (EC50) in milli- (mM) or micromolar concentrations (μM) and Hill coefficients (n) are given to summarize transport activities in comparison to computed binding energies (Eint) of selected hexameric complexes with chloride (Fig. 1b). For original transport data, seeFig. 3a,b, andSupplementary Figs S6–S9). For DFT-optimized hexamers, the point group of symmetry is listed in square parenthesis. Figure 2: Candidates tested for anion transport with halogen bonds. Effective concentrations ( EC 50 ) in milli- (mM) or micromolar concentrations (μM) and Hill coefficients ( n ) are given to summarize transport activities in comparison to computed binding energies ( E int ) of selected hexameric complexes with chloride ( Fig. 1b ). For original transport data, see Fig. 3a,b , and Supplementary Figs S6–S9 ). For DFT-optimized hexamers, the point group of symmetry is listed in square parenthesis. 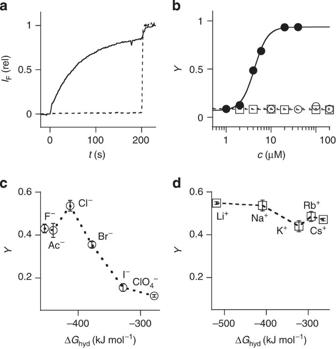Figure 3: Transport activity and ion selectivity in vesicles. (a) Change in ratiometric fluorescence emission intensityIF(λem=510 nm,λex=450/405 nm) as a function of the timet(in secondss) during the addition of 4 (20 μM, 0 s) and excess gramicidin D (200 s) to EYPC vesicles with internal HPTS and externally added NaOH (20 μl, 0.5 M, solid), compared with4(2 mM) added to EYPC vesicles with internal 5(6)-CF (λex=492 nm,λem=517 nm, dashed). (b) Dependence of the fractional transport activityYin the HPTS assay on the concentrationcof5(empty squares),6(filled circles) and7(empty circles). (c) Dependence of the activityYof 15 on the hydration energy ΔGhydof extravesicular anions (100 mM NaX, inside 100 mM NaCl). (d) Same for cations (100 mM MCl, inside 100 mM NaCl). Error bars depict standard errors (s.e.) of at least two independent experiments. Full size image Figure 3: Transport activity and ion selectivity in vesicles. ( a ) Change in ratiometric fluorescence emission intensity I F ( λ em =510 nm, λ ex =450/405 nm) as a function of the time t (in seconds s ) during the addition of 4 (20 μM, 0 s) and excess gramicidin D (200 s) to EYPC vesicles with internal HPTS and externally added NaOH (20 μl, 0.5 M, solid), compared with 4 (2 mM) added to EYPC vesicles with internal 5(6)-CF ( λ ex =492 nm, λ em =517 nm, dashed). ( b ) Dependence of the fractional transport activity Y in the HPTS assay on the concentration c of 5 (empty squares), 6 (filled circles) and 7 (empty circles). ( c ) Dependence of the activity Y of 15 on the hydration energy Δ G hyd of extravesicular anions (100 mM NaX, inside 100 mM NaCl). ( d ) Same for cations (100 mM MCl, inside 100 mM NaCl). Error bars depict standard errors (s.e.) of at least two independent experiments. Full size image As an experimental model of the anion-binding abilities of the iodoperfluoroalkyl transporters, we decided to co-crystallize 18-crown-6 (1,4,7,10,13,16-hexaoxacyclooctadecane) with potassium chloride (KCl), and nonafluoro-1-iodobutane 4 . The single-crystal X-ray structure of the obtained ternary co-crystal revealed that two perfluorobutyl iodide molecules bind tightly to the same chloride anion (Cl − ...I distance=3.040(1) Å, corresponding to an ~20% reduction of the sum of van der Waals and Pauling ionic radii for I and Cl − (ref. 26 ), respectively; Cl − ...I-C angle=177.54(2)° and I...Cl − ...I angle=118.06(1)°) ( Fig. 1d ). The coordination sphere of the chloride anion is completed by two potassium cations (K + ...Cl − distance=3.298(1) Å), which, in turn, are included into two different crown ether molecules ( Supplementary Figs S1 and S2 ). 18-Crown-6 KI also crystallizes as a hydrate ( Supplementary Fig. S3 ) [27] , but in the presence of heptafluoro-1-iodopropane 3 , a 1:2 co-crystal is formed wherein the transporter 3 , that is, halogen bonds, substitutes for water, that is, hydrogen bonds ( Supplementary Figs S4 and S5 ; Supplementary Tables S1 and S2 ). This ternary co-crystal is strictly isostructural with 18-crown-6 KI/ 4 co-crystal, indicating how robust the anion-iodoperfluorocarbon supramolecular synthon is. The binding of more transporters, as predicted from theory ( Fig. 1e ) and transport experiments (below), was hindered in the co-crystals by the presence of the bulky 18-crown-6-complexed counterions. Although the situation in the solid state differs from transport in membranes, the obtained structures confirm that at least two strong halogen bonds do occur between iodoperfluoroalkyl transporters and halide anions. Transport activity The activity of the nineteen candidates 1 - 19 was evaluated first with the 8-hydroxy-1,3,6-pyrenetrisulfonate (HPTS) assay ( Fig. 3 ) [25] . In this assay, large unilamellar vesicles composed of egg yolk phosphatidylcholine (EYPC LUVs) are loaded with the pH-sensitive fluorophore HPTS, and a transmembrane pH gradient is applied. After the addition of transporters such as perfluoro-1-iodobutane 4 , the velocity of pH gradient collapse was followed by ratiometric fluorescence kinetics ( Fig. 3a , solid, Supplementary Figs S6–S8 ). The dose-response curve revealed the effective concentration EC 50 =21.6 μM and the Hill coefficient n =4.7 for the minimalist transporter 4 ( Figs 2 and 3a ; Supplementary Fig. S9 ; Supplementary Table S3 ). The EC 50 is related to the dissociation constant K D of the active complex [25] , whereas the Hill coefficient n can describe the number of monomers in the active complex; thermodynamically stable systems give underestimates [25] , [28] . Hill coefficients up to 4.7 were consistent with computational results for halogen-bonded capsules as active structures for hydroxides ( Figs 1 and 2 ). In contrast, the inability of up to 2 mM iodobutane 4 to transport the much larger 5(6)-carboxyfluorescein (CF) demonstrated that leakage-free activity is recorded in the HPTS assay ( Fig. 3a , dashed; Supplementary Fig. S10 ). The highest activity was observed for perfluoroiodohexane 6 ( EC 50 =3.07±0.15 μM; Fig. 2 and 3b , filled circles). Shorter linear perfluoroiodoalkanes showed decreasing activity. Molecular models indicated that trifluoromethyl or linear heptafluoropropyl tails are too short to fully encapsulate chloride anions ( Fig. 1b ). Poor partitioning of such complexes in lipid bilayers could thus account for the loss in activity. Moreover, the formation of larger, transport-active bundles within the lipid bilayer should also be less effective. Higher activity of the iso -iodopropane 2 with EC 50 =30.0 μM was consistent with improved anion encapsulation by branched fluoroalkyl tails. This interpretation was in agreement with molecular models. Exposure of the entire transport system to heat (60 °C) before and during the experiment did not change significantly the activity of transporter 2 (bp=39 °C; Fig. 4c , filled circles). However, transporter 2 evaporated rapidly when a nitrogen flow was applied during the initial heating ( Fig. 4c , empty circles). Reduction of activity due to flow-mediated evaporation at 60 °C was more pronounced above the boiling point of 2 ( Fig. 4c , empty circles) than below the boiling point of 6 (bp=117 °C; Fig. 4c , empty squares; Supplementary Fig. S11 ). Relatively poor, yet detectable activity observed for trifluoroiodomethane 1 (bp=−22 °C) was consistent with the observed trends for decreasing anion encapsulation ( Fig. 2 ). Bubbling of the gas 1 at a flow rate of 30 ml min −1 through an aqueous suspension of HPTS-loaded LUVs before triggering the transport measurements with a base pulse turned on anion transport activity with an effective bubbling time of 39±4 s ( Fig. 4a,b ). 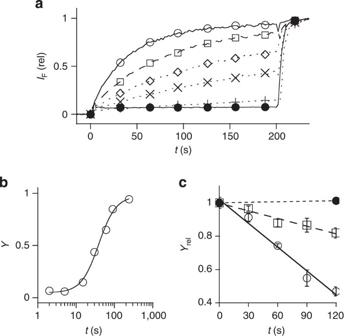Figure 4: Addition and elimination of volatile transporters. (a) Activity in the HPTS assay after bubbling1(empty symbols, with increasing activity, 15, 30, 60, 90 and 240 s; 30 ml min−1) or N2(filled circles, 30 min) through the suspension of EYPC vesicles. Activity is measured as ratiometric change in fluorescence emission intensityIF(λem=510 nm,λex=450/405 nm) as a function of timetduring the addition of NaOH (20 μl, 0.5 M) and excess gramicidin D (200 s). (b) Fractional transport activityYof1, as a function of the timet, the gas was bubbled through the assay suspension before measurements (froma). (c) Relative fractional activityYrelof2(30 μM, circles) and6(4 μM, squares) as a function of incubation timetat 60 °C before the application of the pH gradient, with (empty symbols) and without (filled symbols) N2flux through the cuvette (0.2 ml s−1). Error bars depict s.e. of at least two independent experiments. Figure 4: Addition and elimination of volatile transporters. ( a ) Activity in the HPTS assay after bubbling 1 (empty symbols, with increasing activity, 15, 30, 60, 90 and 240 s; 30 ml min −1 ) or N 2 (filled circles, 30 min) through the suspension of EYPC vesicles. Activity is measured as ratiometric change in fluorescence emission intensity I F ( λ em =510 nm, λ ex =450/405 nm) as a function of time t during the addition of NaOH (20 μl, 0.5 M) and excess gramicidin D (200 s). ( b ) Fractional transport activity Y of 1 , as a function of the time t , the gas was bubbled through the assay suspension before measurements (from a ). ( c ) Relative fractional activity Y rel of 2 (30 μM, circles) and 6 (4 μM, squares) as a function of incubation time t at 60 °C before the application of the pH gradient, with (empty symbols) and without (filled symbols) N 2 flux through the cuvette (0.2 ml s −1 ). Error bars depict s.e. of at least two independent experiments. Full size image Elongation of the perfluoroalkyl tails up to iodododecane 12 caused inactivity ( Fig. 2 ). Possibly, these longer tails prefer to align with the lipid tails in the bilayer membrane. Such an alignment would be incompatible with spherical anion complexes that can move across the membrane. Alternatively, the increasingly hydrophobic transporters could aggregate and precipitate before partitioning into the bilayer. The sharp transition from highest activity with hexyl and inactivity with octyl tails confirmed that highly cooperative processes, possibly including the higher order self-assembly into bundles, are needed for transport. In any case, decreasing activity with increasing tail length clearly disfavoured defects along co-axial fluoroalkyl and lipid tails as active structures ( Fig. 1b,c ). Inactivity with defluorinated iodohexane 5 and deiodinated perfluorohexane 7 demonstrated that the activity of perfluorinated iodohexane 6 originates from halogen bonding ( Fig. 3b , empty symbols). Exactly the same trends were observed for arene transporters. Namely, the moderate activity of pentafluoroiodobenzene 9 faded steadily in perfluorinated bromobenzene 11 , defluorinated iodobenzene 18 , and benzene 19 ( Fig. 2 ). The good correspondence of activities with computed stabilities indicated that the active complexes remain too unstable to enter the inhibitory regime, known to cause decreasing activity when anions are bound too strongly and release is becoming too slow [13] , [29] . This interpretation was further supported by the high Hill coefficients, because the Hill equation applies only to thermodynamically less stable suprastructures with monomers in excess, whereas exergonic self-assemblies give n ~1 (refs 25 , 28 ). Inactive were hexafluorobenzene 13 as homologous probe for anion-π interactions [10] , [11] , perfluorophenol 14 as probe for hydrogen bonds, and diiodopyridinium 17 as probe for symport, the latter two, possibly, also because of their high hydrophilicity. Increased effective halogen-bond donor concentrations made the divalent diiodoarenes 15 and 16 the most active aromatic transporters. Ion selectivity and voltage dependence Ion selectivities were first determined by external ion exchange in the HPTS assay. Insensitivity to cation exchange suggested that cations are not involved in transport ( Fig. 3d ). In contrast, the activity of perfluorinated o -diiodobenzene 15 decreased significantly with decreasing dehydration penalty of anions ( Fig. 3c ; Supplementary Figs S12 and S13 ). This quasi anti-Hofmeister sequence Cl − >Br − >I − confirmed predictions from theory that the cost of dehydration will be overcompensated by binding. All these results implied the occurrence of a clean, cation-independent anion antiport. The addition of transporters such as iodobenzene 9 caused a steady increase in current across black lipid membranes (BLM) ( Fig. 5a ). The absence of measurable step conductance changes was consistent with a carrier-type ion transport mechanism. The current–voltage ( I – V ) dependence of 9 was clearly nonlinear ( Fig. 5c ). Exponential curve fit gave a formal [25] gating charge z g =0.41. Similarly, high values were observed for 4 ( z g =0.42) and 15 ( z g =0.41, Supplementary Figs S14 and S15 ; Supplementary Table S4 ). The significant voltage dependence of transporters with halogen bonds can be explained by the mechanism proposed for the biological carrier monactin, in which the rate-limiting transmembrane ion transport is accelerated by the applied voltage [30] . However, alternative explanations, such as changes in diffusion length on membrane thinning at high voltage, deserve consideration, and the possible role of counterions under these conditions remains to be clarified [31] . 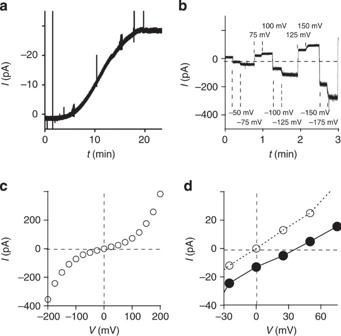Figure 5: Voltage dependence and ion selectivity in planar bilayer conductance experiments. (a) CurrentIin picoamperes pA in BLMs as a function of timetafter the addition of9(500 μM) to thecischamber, applied voltageV=−50 mV, 2 M KClcisandtrans. (b) CurrentIin BLMs as a function of timetin the presence of9(500 μMcis), applied voltage −200 mV ≤V≤+200 mV, 2 M KClcis, 1 M KCltrans. (c) Dependence of the currentIon the applied voltageVin the presence of9(500 μMcis), 2 M KClcisandtrans. (d)I-Vprofile, 2 M KClcisandtrans(empty circles) or 2 M KClcisand 0.25 M KCl intrans(filled circles). Figure 5: Voltage dependence and ion selectivity in planar bilayer conductance experiments. ( a ) Current I in picoamperes pA in BLMs as a function of time t after the addition of 9 (500 μM) to the cis chamber, applied voltage V =−50 mV, 2 M KCl cis and trans . ( b ) Current I in BLMs as a function of time t in the presence of 9 (500 μM cis ), applied voltage −200 mV ≤V≤+200 mV, 2 M KCl cis , 1 M KCl trans . ( c ) Dependence of the current I on the applied voltage V in the presence of 9 (500 μM cis ), 2 M KCl cis and trans . ( d ) I-V profile, 2 M KCl cis and trans (empty circles) or 2 M KCl cis and 0.25 M KCl in trans (filled circles). Full size image Application of salt gradients resulted in an asymmetric response to voltage ( Fig. 5b ). Permeability ratios were calculated from reversal potentials using the Goldman–Hodgkin–Katz equation ( Fig. 5d ; Supplementary Figs S14 and S15 ; Supplementary Table S4 ). Permeability ratios up to P Cl−/K+ =37.1 for iodobutane 4 were found. Iodoaryl transporters 9 and 15 gave lower but still highly significant selectivities (both P Cl−/K+ =9.9). These permeability ratios demonstrated that the anion/cation selectivity of iodoalkyl transporters is exceptional; anion channels are usually around P Cl−/K+ ~5 (ref. 32 ). Membrane composition and additives According to the HPTS assay, activities in the anionic EYPG (egg yolk phosphatidylglycerol) LUVs were about one order of magnitude below those in the zwitterionic EYPC LUVs ( Supplementary Figs S16 and S17 ; Supplementary Table S3 ). This result was consistent with the proposed translocation mechanism. The proposed active supramolecule is overall negatively charged and has an electronegative surface ( Fig. 1b,c ). Reduced activity on charge repulsion between anionic vesicles and anionic transporters supported occurrence of anion antiport without significant contributions from cations. The temperature dependence of anion transport in DPPC (dipalmitoyl phosphatidylcholine) vesicles showed that, by decreasing the fluidity of the membrane, the transport is increasingly hindered ( Fig. 6a,b ; Supplementary Figs S18–S23 ; Supplementary Table S5 ). This observation can be indicative of a carrier mechanism. Interestingly, perfluoro-1-iodobutane 4 was sensitive not only to the main phase transition of DPPC LUVs at 41 °C (ref. 33 ). For DPPC in the pseudocrystalline phase L c′ at T =15 °C, anion transport was almost completely inhibited. With subtransition into the crystalline gel phase L β′ at 19 °C, anion transport became detectable but was still low ( Fig. 6a,b ). After pretransition into the rippled phase P β′ , anion transport further improved to finally reach 'full' activity after the main transition into the fluid phase L α (above 41 °C for DPPC, the same phase as EYPC at 25 °C). The phase transitions can be identified as sharp decreases in the temperature dependence ( Fig. 6b ). In fluid phase, the changes in temperature had little effect in the transport activity, which is consistent with the hypothesis that the observed changes originated from the differences in the membrane structure. 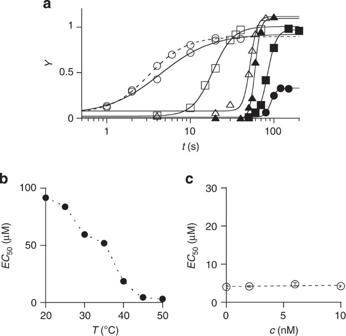Figure 6: Dependence of activity on temperature in DPPC vesicles and on the presence of valinomycin in EYPC vesicles. (a) Dependence of the fractional transport activityYin the HPTS assay on the concentrationcof4in DPPC vesicles at 20 °C (filled circles), 25 °C (filled squares), 30 °C (filled triangles), 35 °C (empty triangles), 40 °C (empty squares), 45 °C (empty circles, solid), 50 °C (empty circles, dashed); for original data, seeSupplementary Figs S18–S23. (b) Dependence of the effective concentrationEC50of4in DPPC vesicles with internal HPTS on the temperatureT; from (a). (c) Dependence of theEC50of6in EYPC vesicles with internal HPTS on the concentrationcof valinomycin, for original data, seeSupplementary Figs S24–S26. Error bars depict s.e. of at least two independent experiments. Figure 6: Dependence of activity on temperature in DPPC vesicles and on the presence of valinomycin in EYPC vesicles. ( a ) Dependence of the fractional transport activity Y in the HPTS assay on the concentration c of 4 in DPPC vesicles at 20 °C (filled circles), 25 °C (filled squares), 30 °C (filled triangles), 35 °C (empty triangles), 40 °C (empty squares), 45 °C (empty circles, solid), 50 °C (empty circles, dashed); for original data, see Supplementary Figs S18–S23 . ( b ) Dependence of the effective concentration EC 50 of 4 in DPPC vesicles with internal HPTS on the temperature T ; from ( a ). ( c ) Dependence of the EC 50 of 6 in EYPC vesicles with internal HPTS on the concentration c of valinomycin, for original data, see Supplementary Figs S24–S26 . Error bars depict s.e. of at least two independent experiments. Full size image Activities in EYPC vesicles were independent of the presence of valinomycin ( Fig. 6c ; Supplementary Figs S24–S26 ). This result provided corroborative evidence for the occurrence of a cation-independent anion antiport. In a system with a transporter that does not operate under an antiport regime, the neutrality of the system has to be maintained by a quasi-simultaneous cation transport. If the cation transport limits the overall rate of transport, the addition of a specific cation transporter, in this case the potassium-selective valinomycin, should lead to significant increase in activity with increasing concentration [34] . In the present case, no significant increase in activity was observed ( Fig. 6c ), indicating that contributions from cation transport are indeed irrelevant. This conclusion was consistent with the results for ion selectivity in EYPC vesicles, poor activity in anionic vesicles, and with very high anion/cation permeability ratios in conductance experiments. The expansion of the number of interactions available to create new functional systems is of paramount importance. Here we provide experimental evidence that halogen bonding can be added to the interactions capable to mediate the transport of anions across lipid bilayers, that is, hydrogen bonding, ion pairing, anion-macrodipole and anion-π interactions. Strong and directional, halogen bonds are best considered as hydrophobic equivalents of hydrogen bonds. Anion transporters that work with halogen bonds can thus be very small, and their boiling point can be very low. The arguably most spectacular expression of these unique characteristics, reported in this study, is that trifluoroiodomethane, a highly volatile compound with a boiling point of −22 °C, can transport anions across lipid bilayer membranes. With one carbon only, this is the smallest possible organic ion transporter. Molecular models, crystal structures and structure-activity relationships are consistent with a general active structure composed of up to six halogen-bond donors surrounding the anion in quasi-octahedral geometry. This structural motif is not novel but sufficient to explain all observed trends. For instance, increasing activity from the fairly modest activity of trifluoroiodomethane to maximal activity with perfluorohexyl tails can be rationalized with increasing thickness and compactness of the hydrophobic shell around the anion. In general, the absolute activities expressed in EC 50 's are comparably poor, which is not further surprising, considering the implication from Hill analysis that, at least, penta- to hexameric active structures represent a minority population with the majority coexisting as inactive monomers [25] , [28] . Previous efforts to reduce size and sophistication have sometimes lead to 'poorly behaved' ion transport systems (that is, detergent effects, poor responsiveness to physical or chemical stimulation, and so on) [1] , [2] , [4] , [12] , but not so with halogen bonds. The characteristics of anion transport mediated by halogen bonds are surprisingly clean and interesting, despite the small size and poor sophistication of the explored systems. Highlights include the absence of nonspecific leakage and the presence of high cooperativity, high voltage dependence and high anion selectivity. The superb properties of anion transporters with halogen-bond donors are attractive for applications reaching from the materials to the life sciences. Direct impact is expected for the design of innovative transport, sensing and delivery systems. The successful delivery of a gas indicates that administration of new transporters to the lungs by inhalation could be of interest for medicinal purposes [3] , [4] . Considering the impressive behaviour of small systems without sophistication, one might wonder what could be obtained when engineering halogen bonds into more refined architectures such as artificial or biological β-barrels [1] , [2] . Broader perspectives include applications to the design of drugs and probes that can enter cells more easily, compact organocatalysts that stabilize anionic transition states also in highly nonpolar solvents or lipid bilayer membranes, or advanced functional materials without complications from hydrophilic recognition motifs. Materials Reagents for synthesis, analysis and crystals were purchased from Fluka, Sigma-Aldrich or Apollo Scientific, buffers and salts of the best grade available from Fluka or Sigma-Aldrich and used as received. 2,5-Diiodo-1-methylpyridin-1-ium iodide ( 17 ) was freshly synthesized ( Supplementary Fig. S27 ). HPTS was from Fluka. EYPC, EYPG, DPPC and a Mini-Extruder used for vesicle preparation were from Avanti Polar Lipids. Fluorescence measurements were performed with a FluoroMax-4 spectrofluorometer (Horiba) equipped with a stirrer and a temperature controller; all measurements were performed at 25 °C unless specified [7] , [11] . Currents were recorded at different holding potentials ( trans at ground) in a house-made Faraday cage, amplified (BC-525c, Warner Instrument), low-pass filtered with an 8-pole Bessel filter at 1-5 kHz (LPF-8, Warner), A-D converted (DigiData 1200, Axon Instruments), and sampled at 10 kHz by computer (pClamp 8.0, Axon) [35] . If necessary, the data were further filtered using pClamp 8.0 or Origin (version 7, OriginLab). All the conductance measurements were performed at room temperature (22±1 °C). X-ray analysis was done on a Bruker KAPPA APEX II diffractometer. The X-ray generator was operated at 50 kV and 30 mA using Mo-Kα radiation. Data were collected with ω and scan with the scan width 0.5. The sample to detector distance was fixed at 40 mm. RLATT was used for sorting of reflections and indexing. The data were reduced with empirical absorption correction. Vesicle preparation EYPC-LUVs HPTS were prepared following established procedures [7] , [11] , [35] . A thin lipid film was prepared by evaporating a solution of 25 mg EYPC in 2 ml MeOH/CHCl 3 (1:1) on a rotary evaporator (40 °C) and then in vacuo overnight. After hydration (>30 min) with 1.0 ml buffer (100 mM NaCl, 10 mM Hepes, 5 mM Na 2 O 3 S 2 , 1 mM HPTS, pH 7.0), the resulting suspension was subjected to >5 freeze-thaw cycles (liquid N 2 , 37 °C water bath) and >15 times extruded through a polycarbonate membrane (pore size 100 nm, Avanti). Extravesicular components were removed by size-exclusion chromatography (Sephadex G-50, Sigma-Aldrich) with 100 mM NaCl, 10 mM Hepes, 5 mM Na 2 O 3 S 2 , pH 7.0. Final conditions: ~2.5 mM EYPC; inside: 100 mM NaCl, 10 mM Hepes, 5 mM Na 2 O 3 S 2 , 1 mM HPTS, pH 7.0; outside: 100 mM NaCl, 10 mM Hepes, 5 mM Na 2 O 3 S 2 , pH 7.0. DPPC-LUVs HPTS, EYPG-LUVs HPTS and EYPC-LUVs CF were prepared analogously ( Supplementary Figs S11 , S16–23 ). Ion transport in vesicles In a typical experiment [7] , [11] , [35] , EYPC-LUVs HPTS (25 μl, final lipid concentration ~31.3 μM) were added to gently stirred, thermostated buffer (1.930 ml; 100 mM NaCl, 10 mM Hepes, 5 mM Na 2 O 3 S 2 , pH 7.0; 25 °C, or as indicated) in a disposable plastic cuvette. Fluorescence emission was followed at λ em =510 nm ( λ ex =450/405 nm) during the addition of first 0.5 M NaOH (20 μl) and then transporter (40 μl stock solution, usually in MeOH) or vice versa , and excess gramicidin D at the end (20 μl, 100 μM in DMSO). Time courses of fluorescence intensity I F were obtained by ratiometric analysis ( R = I t,450 / I t,405 ) and normalization according to equation (1) where R 0 = R t right before the addition of transporter and R ∞ = R t after addition of gramicidin D ( Fig. 3a , solid; Supplementary Figs S6–S8 ). I F at 300 s, just before addition of gramicidin D, was defined as fractional activity Y , and analysed with the Hill equation (2) to give effective concentration EC 50 and the Hill coefficient n , where Y 0 is Y in absence of transporter , Y ∞ is Y with excess transporter, and c is the transporter concentration in the cuvette ( Fig. 3b ; Supplementary Fig. S9 ). Complete results for all compounds are shown in Fig. 2 and Supplementary Table S3 . The experiments with DPPC-LUVs HPTS ( Fig. 6a,b ; Supplementary Figs S18–S23 ; Supplementary Table S5 ) and EYPG-LUVs HPTS ( Supplementary Figs S16, S17 ; Supplementary Table S3 ) followed the same procedure using different vesicle stock solutions. Gaseous transporter 1 was also added by bubbling through the vesicles suspension for 15–240 s before the addition of base (at t =0 in Fig. 4a ). To remove volatile transporters, an N 2 flux was applied for increasing times at various temperatures directly before measurement (0–120 s, Fig. 4c ). Transport in the presence of valinomycin ( Fig. 6c ; Supplementary Figs S24-S26 ) and membrane potentials ( Supplementary Figs S28 and S29 ; Supplementary Table S3 ), and ion selectivity experiments by external ion exchange ( Fig. 3c,d ; Supplementary Figs S12 and S13 ) were performed analogously with the HPTS assay. Voltage clamp experiments Conductance experiments in black lipid membranes (BLMs) were performed following established procedures [25] , [35] . BLMs were formed by painting a solution of EYPC in n -decane (42 mg ml −1 ) on an aperture (150 μm, pretreated with EYPC/decane, 42 mg ml −1 ) in a delrin cuvette separating two chambers containing 1 ml each of 0.25 to 2 M KCl and an agar bridge connection (2 M KCl; 2% Agar) to Ag/AgCl electrodes. The transporters were added to the cis chamber at negative holding potential. Formal gating charges were determined from I – V profiles using equation (3) where I =current (pA); z g =gating charge; e =elemental charge; V =applied potential (volt); k =Boltzmann constant; T =temperature (K) ( Fig. 5c ; Supplementary Figs S14 and S15 ; Supplementary Table S4 ). Salt gradients were applied to determine the ion selectivities. Chloride vs potassium permeability ratios P C l - / P K + were calculated from the reversal potentials V r obtained under KCl concentration gradients using the equation derived from Goldman–Hodgkin–Katz voltage equation (4). where P C l - / P K + = anion/cation permeability ratio; a K + c i s = potassium activity in the cis chamber; a K + t r a n s = potassium activity in the trans chamber; a C l - c i s = chloride activity in the cis chamber; a C l - t r a n s = chloride activity in the trans chamber; Vr=reversal potential; F=Faraday constant; R=gas constant; T =temperature (K) ( Fig. 5b,d , Supplementary Figs S14 and S15 ; Supplementary Table S4 ). Computational studies The geometries of halogen-bonded complexes were optimized at the M06-L/6-311G** level of theory [23] , using the Gaussian 09 program [36] . For iodine, the basis set was taken from the EMSL Basis Set Exchange website [37] . At the beginning of the optimization for each halogen-bonded complex, the highest possible symmetry was imposed. To verify that the symmetric structure corresponds to minima, vibrational analysis was performed at the same level of theory as the optimization. If the structure obtained was not true minima (one or more imaginary frequencies (NIMEG)), the symmetry point group was lowered and the complex was re-optimized. This strategy was used until the localization of a true minimum (no imaginary frequencies) was confirmed for each complex. The same methodology was followed for the optimization of complexes between the perfluoro-1-iodobutane 4 and the chloride anion (Cl − ) or the hydroxide anion (OH − ) at various stoichiometries. The interaction energies were computed at the M06-2X/6-311G**//M06-L/6-311G** level of theory [24] and corrected for the basis set superposition error using the counterpoise method. Crystal structures 1,4,7,10,13,16-Hexaoxacyclooctadecane (18-crown-6) and perfluoroiodoalkanes, were used without further purification. Potassium chloride or potassium iodide (KCl/KI) was used after drying for 2 h at 433 K. A 1:1 mixture of 18-crown-6 and KCl or KI were stirred in the presence of excess amount of iodoperfluoroalkane (50 eq). Then, the system was heated to the boiling point of perfluoroiodoalkane in a vial for a few minutes. After allowing for slow cooling at room temperature, the complex 18-crown-6 KI heptafluoro-(1-iodopropane) 2 was isolated as plate-shaped crystals after the solution was maintained at room temperature for, 3 h. The complex 18-crown-6 KCl (nonafluoro-1-iodobutane) 2 formed as plate-shaped crystals after 5 days at 4 °C. Crystal selection was made under polarized light microscope. A single crystal was chosen for X-ray analysis and the data were collected at 100(2) K using liquid nitrogen cryo-system to avoid the evaporation of the perfluoro-1-iodoalkane. Structures were solved by direct method using SHELXL97 (ref. 38 ) present in the program suite WinGX (version 1.80.04) [39] . The molecular diagrams were generated from ORTEP and the packing diagrams were generated using Mercury. Geometrical calculations were done using PARST95 and PLATON. The non-hydrogen atoms are refined anisotropically and hydrogen atoms were refined using difference Fourier map or positioned geometrically. All crystallographic details are listed in the Supplementary Table S1 , and intermolecular interactions are listed in the Supplementary Table S2 . Crystallographic data is provided as Supplementary Data 1 , 2 , 3 . IR (infrared, selected peaks): 18-crown-6 (solid), 3501, 2866, 1721, 1451, 1315, 1295, 1250, 1108, 989, 947, 843; nonafluoro-1-iodobutane (liquid), 1346, 12356, 1199, 1138, 1091, 993, 950, 850, 852, 792, 744, 716, 682, 630 cm −1 ; heptafluoro-1-iodopropane (liquid): 1330, 1273, 1244, 1226, 1155, 11331066, 1033, 881, 818, 733, 671 cm −1 ; 18-crown-6 KCl (nonafluoro-1-iodobutane) 2 (solid): 1305, 1228, 1182, 1122, 982, 891, 808, 745, 715, 649 cm −1 ; 18-crown-6 KI (heptafluoro-1-iodo-propane) 2 (solid): 3387, 2895, 1721, 1472, 1352, 1328, 1286, 1269, 1222, 1202, 1187, 1105, 1060, 1025, 963, 875, 840, 811, 729, 666 cm −1 . Accession codes: CCDC 867713 , 867714 , and 867716 contain the supplementary crystallographic data for this paper. These data can be obtained free of charge from The Cambridge Crystallographic Data Centre via www.ccdc.cam.ac.uk/data_request/cif . How to cite this article: Jentzsch, A. V. et al . Transmembrane anion transport mediated by halogen-bond donors. Nat. Commun. 3:905 doi: 10.1038/ncomms1902 (2012).